Co-operativity in a nanocrystalline solid-state transition Co-operativity is a remarkable phenomenon mostly seen in biology, where initial reaction events significantly alter the propensity of subsequent reaction events, giving rise to a nonlinear tightly regulated synergistic response. Here we have found unique evidence of atomic level co-operativity in an inorganic material. A thousand-atom nanocrystal (NC) of the inorganic solid cadmium selenide exhibits strong positive co-operativity in its reaction with copper ions. A NC doped with a few copper impurities becomes highly prone to be doped even further, driving an abrupt transition of the entire NC to the copper selenide phase, as manifested by a strongly sigmoidal response in optical spectroscopy and electron diffraction measurements. The examples presented here suggest that cooperative phenomena may have an important role in the solid state, especially in the nucleation of new chemical phases, crystal growth, and other materials’ transformations. Since the first observation in 1910 of the co-operative binding of oxygen to haemoglobin [1] , [2] , where binding at any of the four sites of haemoglobin increases the oxygen affinity of the other sites, co-operative phenomena have been displayed in a host of macromolecular systems [3] , ranging from the unwinding of DNA and protein folding [4] to self-assembly in supramolecular systems [5] . A common feature of co-operative systems is that they possess multiple binding sites with some mechanism for feedback or coupling between the binding sites. The feedback itself may be positive or negative. Positive co-operativity is manifested as an apparent all-or-nothing behaviour [6] : rather than making a gradual progression through intermediary states, the system undergoes a relatively abrupt transition from the initial to the final state in response to an extremely small change in conditions (for example, ligand, denaturing agent, pH or temperature). The system spends little time in the intermediary states, resulting in their low population. The strongly sigmoidal oxygen-binding curve of haemoglobin is the archetypal example of such behaviour [1] . Although examples of co-operativity seem limited to macromolecules, mostly biological [3] , we found evidence of co-operative behaviour in an inorganic solid material. The observation was made in nanocrystals (NCs) of cadmium selenide (CdSe) [7] undergoing a cation exchange in the presence of monovalent ions as: In this transformation [8] , [9] , the Cd 2+ cationic sub-lattice is replaced with Cu + ions, two for every Cd 2+ ion, to form a NC of cuprous selenide (Cu 2 Se). Each CdSe NC is ∼ 4 nm or ∼ 1,300 atoms in size, and loosely speaking, can be thought of as a ‘macromolecular system’ with multiple ‘sites’ for foreign cations. The cation exchange reaction [10] itself has received a lot of fundamental attention because of its remarkably fast (millisecond timescale) kinetics [11] in nanosized crystals. The transformation, if well understood, can be exploited for topotaxially templated synthesis of nanostructures with novel compositions and morphologies [12] , [13] , designing heterojunctions in NCs [14] , sensing heavy metal ions [15] , and achieving electronic doping [16] , [17] . With limited mechanistic insight available, cation exchange is often assumed to be a diffusion-limited transformation: as long as the cation can diffuse to a lattice site, exchange can take place at that site. By this assumption, all lattice sites exposed to Cu + would have an equal affinity for exchange and the CdSe ensemble would transform in a random site-by-site manner to the Cu 2 Se phase as adequate Cu + becomes available. However, our optical and electron diffraction measurements show that the exchange transformation does not follow such a memoryless, diffusion-limited process. Instead, we see positive co-operative behaviour, where initial Cu + doping of a NC strongly enhances the likelihood of further Cu + doping within the same NC, causing the NC to transition sharply from a lightly doped CdSe NC to the Cu 2 Se phase. Optical probing of cation exchange We used excitonic absorption spectra ( Fig. 1a ) to monitor the cation exchange of a solution of 4-nm CdSe NCs as it was titrated with Cu + . With increasing Cu + feed concentration, the excitonic band at 2.1 eV, corresponding to the 1 S h –1 S e transition in the CdSe NCs, decreased in intensity, which is expected as the conversion to Cu 2 Se proceeded. Concomitantly, the absorption in the near-infrared region associated with Cu 2 Se increased. 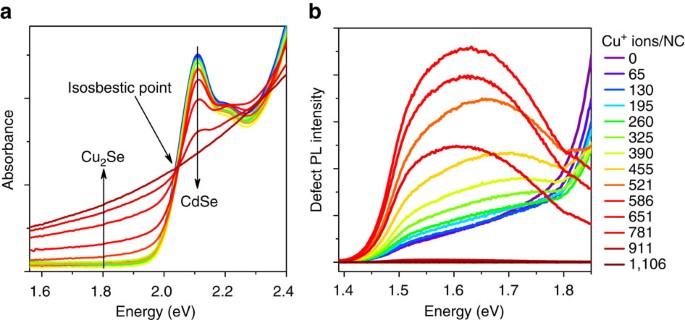Figure 1:Optical monitoring of the cation exchange reaction of CdSe NCs with Cu+. Excitonic absorption spectra (a) of an ensemble of CdSe NCs as a function of added Cu+. Feed Cu+concentrations are denoted as the number of ions available per CdSe NC. With increasing addition of Cu+, the CdSe NC exciton peak at 2.1 eV decreases without undergoing any shift. Concomitantly, the Cu2Se absorption in the near-infrared increases. A clear isosbestic point is seen. Following complete exchange, the absorption spectrum of the NCs resembles that of Cu2Se with a bandgap onset around 1 eV. Note, Cu2Se is an indirect semiconductor and therefore has no excitonic band, rather only a featureless absorption above its bandgap. PL spectra (b) in the sub-bandgap region show the emergence of defect luminescence when Cu+is added, which evolves further with increasing Cu+feed concentration. The excitonic bandgap PL of CdSe NCs was subtracted out from these spectra, as detailed in the Methods section. Figure 1: Optical monitoring of the cation exchange reaction of CdSe NCs with Cu + . Excitonic absorption spectra ( a ) of an ensemble of CdSe NCs as a function of added Cu + . Feed Cu + concentrations are denoted as the number of ions available per CdSe NC. With increasing addition of Cu + , the CdSe NC exciton peak at 2.1 eV decreases without undergoing any shift. Concomitantly, the Cu 2 Se absorption in the near-infrared increases. A clear isosbestic point is seen. Following complete exchange, the absorption spectrum of the NCs resembles that of Cu 2 Se with a bandgap onset around 1 eV. Note, Cu 2 Se is an indirect semiconductor and therefore has no excitonic band, rather only a featureless absorption above its bandgap. PL spectra ( b ) in the sub-bandgap region show the emergence of defect luminescence when Cu + is added, which evolves further with increasing Cu + feed concentration. The excitonic bandgap PL of CdSe NCs was subtracted out from these spectra, as detailed in the Methods section. Full size image Two important features emerge in these spectra. First, the spectral position of the CdSe exciton stayed relatively unchanged throughout the titration, which indicates an absence [13] of any significant fraction of binary CdSe/Cu 2 Se NCs formed by partial cation exchange. Such heterostructures would exhibit strongly shifted excitonic peaks, because the excitonic peak position is highly dependent on the CdSe crystallite size [18] . Although it is possible that partial conversion of a CdSe NC to Cu 2 Se completely quenches its excitonic absorption, this possibility is excluded by a key observation: the decrease in the fraction of CdSe NCs (estimated from the CdSe exciton height) is perfectly correlated with the increase in the fraction of Cu 2 Se NCs (estimated from the Cu 2 Se absorbance at 1.82 eV), as shown in Fig. 2 . A clear isosbestic point ( Fig. 1a ) is identified, which is a well-known indicator of a two species system, where one species converts to another over the course of the titration. Thus, it appears that individual CdSe NCs switch fully to Cu 2 Se as sufficient Cu + becomes available. With increasing amount of Cu + , more and more NCs make this transition from CdSe to Cu 2 Se. Thus, each NC is either in the CdSe state (albeit with some Cu + dopants) or in the fully exchanged Cu 2 Se state, manifesting the classic two-state behaviour of a co-operative system. 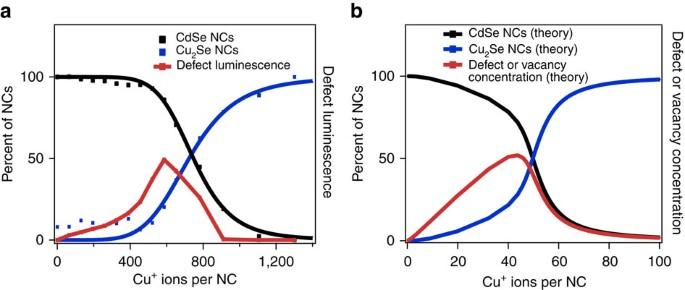Figure 2: Sigmoidal nature of the cation exchange titration. Experimental plot (a) of the fraction of NCs in the CdSe state (black) and those in the Cu2Se state (blue) as a function of added Cu+is strikingly sigmoidal, representative of a strongly co-operative process. Below a critical concentration of∼500 Cu+ions per NC, very few NCs undergo a transition to the Cu2Se state. A fit to the Hill plot (solid black line,R=0.996) yields a co-operativity factor ofnH=7.1. Note we use total Cu+concentration, although the Hill equation is strictly valid for free concentrations. The fraction of NCs in the CdSe state was determined from the height of the CdSe excitonic peak fromFig. 1aand the fraction in the Cu2Se state was determined from the Cu2Se band-to-band absorption at 1.82 eV. The procedure for analysis is described in Methods. The rise in the Cu2Se fraction tracks well with the drop in the CdSe fraction, further confirming two-state behaviour. The defect luminescence intensity (red), integrated across the broad band shown in Fig. 1b increased as Cu+was added, until it reached a maximum around the critical concentration, beyond which it decreased, until it reached zero. A theoretical simulation (b) of a 20-site NC reproduced the observed nature of the cation exchange transformation. Sequential binding was used to model the positive co-operative behaviour. The simulated fraction of Cu2Se NCs in solution as a function of the total Cu+concentration, plotted as the number of ions per NC, follows a strongly sigmoidal curve (blue). The fraction of all NCs in the CdSe state, either pure or doped, is also shown (black). The simulated concentration of Cu+dopants and associated Cd2+vacancies (red) reproduces the observed evolution of the defect luminescence. The defect concentration reaches a maximum around the critical Cu+concentration, beyond which it gradually decreases to zero. Figure 2: Sigmoidal nature of the cation exchange titration. Experimental plot ( a ) of the fraction of NCs in the CdSe state (black) and those in the Cu 2 Se state (blue) as a function of added Cu + is strikingly sigmoidal, representative of a strongly co-operative process. Below a critical concentration of ∼ 500 Cu + ions per NC, very few NCs undergo a transition to the Cu 2 Se state. A fit to the Hill plot (solid black line, R =0.996) yields a co-operativity factor of n H =7.1. Note we use total Cu + concentration, although the Hill equation is strictly valid for free concentrations. The fraction of NCs in the CdSe state was determined from the height of the CdSe excitonic peak from Fig. 1a and the fraction in the Cu 2 Se state was determined from the Cu 2 Se band-to-band absorption at 1.82 eV. The procedure for analysis is described in Methods. The rise in the Cu 2 Se fraction tracks well with the drop in the CdSe fraction, further confirming two-state behaviour. The defect luminescence intensity (red), integrated across the broad band shown in Fig. 1b increased as Cu + was added, until it reached a maximum around the critical concentration, beyond which it decreased, until it reached zero. A theoretical simulation ( b ) of a 20-site NC reproduced the observed nature of the cation exchange transformation. Sequential binding was used to model the positive co-operative behaviour. The simulated fraction of Cu 2 Se NCs in solution as a function of the total Cu + concentration, plotted as the number of ions per NC, follows a strongly sigmoidal curve (blue). The fraction of all NCs in the CdSe state, either pure or doped, is also shown (black). The simulated concentration of Cu + dopants and associated Cd 2+ vacancies (red) reproduces the observed evolution of the defect luminescence. The defect concentration reaches a maximum around the critical Cu + concentration, beyond which it gradually decreases to zero. Full size image Across a range of systems, sigmoidal-binding curves are a definitive manifestation of co-operative behaviour [1] . Figure 2 shows such a curve for the cation exchange process: this plot of the fraction of NCs in the CdSe state as a function of Cu + concentration is strikingly sigmoidal, as also is the plot of the fraction of NCs in the Cu 2 Se state. Only a small to negligible fraction of NCs is exchanged at low Cu + feed concentrations. However, once a critical concentration is reached, a major fraction of NCs switch to the Cu 2 Se state over a narrow concentration window about the critical concentration. The titration curve fits well ( R =0.996) the Hill equation [1] , with a Hill coefficient or co-operativity factor of n H =7.1. As a comparison, strongly co-operative oxygen binding by haemoglobin shows a value of n H =2.3–3.0. We have found some experiment-to-experiment variation in the measured n H (range 4–7). Size/shape/surface-related heterogeneities inherent to NC samples may contribute to such variation. Structural probing of cation exchange Electron diffraction measurements ( Fig. 3 ) provide structural evidence of the sharp onset of the cation exchange process. The initial NC samples show wurtzite CdSe diffraction features, which persist up to a Cu + feed concentration as high as 549 ions per NC ( Table 1 ). Around this Cu + concentration (the half-way point), a significant fraction of NCs undergo a conversion to Cu 2 Se, as indicated by the emergence of diffraction features corresponding to the tetragonal belladoite phase of Cu 2 Se, albeit superimposed on wurtzite diffraction features from the remnant CdSe NCs. With further addition of Cu + , the tetragonal Cu 2 Se diffraction pattern becomes more prominent as additional NCs convert to Cu 2 Se. Concomitantly, the wurtzite CdSe diffraction pattern wanes. Eventually, at about 1,317 Cu + ions per NC (slightly higher than a full stoichiometric amount), only the tetragonal Cu 2 Se diffraction pattern is seen, indicating conversion of all NCs to Cu 2 Se. 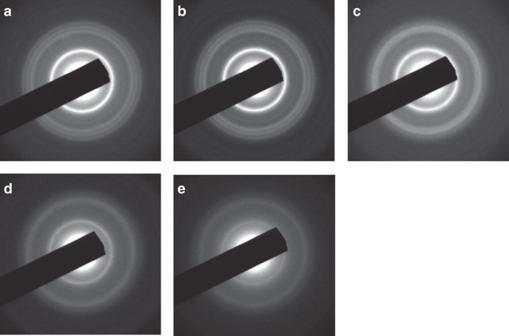Figure 3: Electron diffraction reveals the sharp onset of cation exchange. For NCs subject to 0 Cu+ions per NC and 384 Cu+ions per NC respectively (a,b), selected area electron diffraction patterns are indicative of the CdSe wurtzite (cadmoselite) structure. As shown inTable 1, the innermost ring at 3.55 Å is a combination of the (100), (002) and (101) planes, which are Debye–Scherrer broadened into one ring. The three outer rings, measured at 2.15, 2.00 and 1.88 Å, match those for the (100), (103) and (200) planes of cadmosellite. In addition, there is a ring corresponding to the (102) plane, at a lattice spacing of 2.55 Å. These features are seen for samples (a–c). At 1,317 Cu+ions per NC (in slight excess of the stoichiometric amount needed for full conversion), the tetragonal Cu2Se phase (bellidoite) is seen (e). The highest intensity reflections include ones at 3.46 Å for the (113), (311) and (222) planes, 2.04 Å for the (404) plane, and 1.76 Å for the (226) and (533) plane. The diffraction features of Cu2Se seem to first appear at 549 Cu+ions per NC (c), overlapped with CdSe diffraction features. As exchange progresses, CdSe diffraction features wane, until a pure bellidoite diffraction pattern is obtained for the fully converted sample. All d-spacings are determined relative to the (111) reflection of an Au standard taken under the same conditions. Samples were prepared by a slow titration of CdSe NCs in toluene with increasing amounts of a methanolic solution of Cu+, similar to the titration experiments described in Methods. At various points in the titration, a small aliquot was drop-casted onto an ultrathin carbon transmission electron microscope grid and washed with methanol several times. The total amount of Cu+added is indicated in Table 1 in the form of number of ions per NC, estimated as described in Methods. Figure 3: Electron diffraction reveals the sharp onset of cation exchange. For NCs subject to 0 Cu + ions per NC and 384 Cu + ions per NC respectively ( a , b ), selected area electron diffraction patterns are indicative of the CdSe wurtzite (cadmoselite) structure. As shown in Table 1 , the innermost ring at 3.55 Å is a combination of the (100), (002) and (101) planes, which are Debye–Scherrer broadened into one ring. The three outer rings, measured at 2.15, 2.00 and 1.88 Å, match those for the (100), (103) and (200) planes of cadmosellite. In addition, there is a ring corresponding to the (102) plane, at a lattice spacing of 2.55 Å. These features are seen for samples ( a – c ). At 1,317 Cu + ions per NC (in slight excess of the stoichiometric amount needed for full conversion), the tetragonal Cu 2 Se phase (bellidoite) is seen ( e ). The highest intensity reflections include ones at 3.46 Å for the (113), (311) and (222) planes, 2.04 Å for the (404) plane, and 1.76 Å for the (226) and (533) plane. The diffraction features of Cu 2 Se seem to first appear at 549 Cu + ions per NC ( c ), overlapped with CdSe diffraction features. As exchange progresses, CdSe diffraction features wane, until a pure bellidoite diffraction pattern is obtained for the fully converted sample. All d-spacings are determined relative to the (111) reflection of an Au standard taken under the same conditions. Samples were prepared by a slow titration of CdSe NCs in toluene with increasing amounts of a methanolic solution of Cu + , similar to the titration experiments described in Methods. At various points in the titration, a small aliquot was drop-casted onto an ultrathin carbon transmission electron microscope grid and washed with methanol several times. The total amount of Cu + added is indicated in Table 1 in the form of number of ions per NC, estimated as described in Methods. Full size image Table 1 d-spacings obtained from electron diffraction of NCs at various stages of Cu + exchange. Full size table Cu + doping as a precursor to exchange In the regime below the critical concentration, it is clear that there is little conversion to Cu 2 Se and most of the NCs exhibit the CdSe crystal structure. However, in this regime, the NCs are doped with Cu (1+) impurities, as found from X-ray photoelectron spectroscopy (XPS) ( Fig. 4b,c and Supplementary Fig. S1 ) and elemental analyses ( Supplementary Fig. S2 and Supplementary Table S1 ). Cu + is a common interstitial dopant in CdSe [19] , [20] . It is known that such dopants do not necessarily disrupt the excitonic band or the overall crystallographic structure of CdSe [18] , [19] , which is consistent with our optical and electron diffraction measurements. 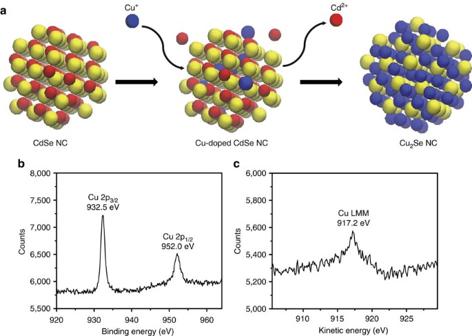Figure 4:Cation exchange is preceded by doping with Cu+. A model of a CdSe wurtzite crystal (a) with ordered cadmium (red) and selenium (yellow) atoms. Below the critical concentration, the CdSe NC uptakes copper ions (blue) in the form of interstitial dopants, in turn creating Cd2+vacancies within the NC for charge compensation. These impurities and vacancies are manifested in the emergence of defect luminescence inFig. 1b. Initial doping events can greatly enhance the affinity of the NC for additional Cu+, eventually triggering a sharp transition to the Cu2Se state. The formation of a Cu2Se NC involves the mutual annihilation of Cu+dopants and Cd2+vacancies, resulting in the decrease in defect luminescence seen above the critical concentration. High-resolution XPS of NCs treated with a copper concentration of 325 Cu+ions per NC are shown (b). NCs were thoroughly washed with methanol to remove excess Cu+before measurements. The fitted peak position of the Cu 2p3/2band (932.5 eV) is indicative of copper ions in the 1+ oxidation state. The Cu LMM peak in the X-ray induced Auger spectrum (c), used to differentiate between Cu+and Cu0, shows a fitted peak position of 917.2 eV, characteristic of Cu(1+). Additional XPS data are shown in theSupplementary Information. Figure 4: Cation exchange is preceded by doping with Cu + . A model of a CdSe wurtzite crystal ( a ) with ordered cadmium (red) and selenium (yellow) atoms. Below the critical concentration, the CdSe NC uptakes copper ions (blue) in the form of interstitial dopants, in turn creating Cd 2+ vacancies within the NC for charge compensation. These impurities and vacancies are manifested in the emergence of defect luminescence in Fig. 1b . Initial doping events can greatly enhance the affinity of the NC for additional Cu + , eventually triggering a sharp transition to the Cu 2 Se state. The formation of a Cu 2 Se NC involves the mutual annihilation of Cu + dopants and Cd 2+ vacancies, resulting in the decrease in defect luminescence seen above the critical concentration. High-resolution XPS of NCs treated with a copper concentration of 325 Cu + ions per NC are shown ( b ). NCs were thoroughly washed with methanol to remove excess Cu + before measurements. The fitted peak position of the Cu 2p 3/2 band (932.5 eV) is indicative of copper ions in the 1+ oxidation state. The Cu LMM peak in the X-ray induced Auger spectrum ( c ), used to differentiate between Cu + and Cu 0 , shows a fitted peak position of 917.2 eV, characteristic of Cu (1+) . Additional XPS data are shown in the Supplementary Information . Full size image Cu + doping can, however, cause lattice defects: for instance, for every two interstitial Cu + impurities in a NC, charge compensation would require the formation of a Cd 2+ vacancy. Both Cu + impurities and vacancies serve as mid-gap trap states and give rise to sub-bandgap luminescence [21] , [22] , [23] , [24] , which we employed for monitoring the doping of NCs at various stages in the cation exchange titration ( Fig. 1b ). Whereas pure CdSe NCs show no sub-bandgap luminescence, addition of Cu + induces a broad defect luminescence in the sub-bandgap 1.4–1.8 eV region. With increasing Cu + feed concentration, the defect luminescence increased in intensity, as would be consistent with an increase in copper impurities and associated defects prior to the onset of cation exchange. The defect luminescence intensity reached a maximum around the critical Cu + concentration, beyond which it started decreasing. Such a decrease is expected from the sharp onset of cation exchange, because the transition to Cu 2 Se involves mutual annihilation of Cu + impurities with Cd 2+ vacancies, expressed in Kroger–Vink notation as: Thus, doping of a CdSe NC with Cu + appears to be a critical precursor to the onset of cation exchange ( Fig. 4a ). The strongest affirmation comes from two observations in Fig. 2a : first, the point in the titration where the defect luminescence intensity reaches a maximum is coincident with the point of onset of cation exchange. Second, the plot of defect luminescence intensity as a function of feed Cu + concentration resembles the derivative of the sigmoidal titration curve. The extended latent region below the critical concentration suggests that the initial incorporation of Cu + into the lattice is a relatively low-probability process. However, initial doping of a NC can occur stochastically, possibly at surface or defect sites of a NC. These initial doping events activate the NC for further doping. Each doping event enhances the affinity of the NC for a subsequent doping event and so on, until the NC reaches a critical state where it is likely to take up every available Cu + ion, resulting in a cascade of Cu + incorporation and an abrupt phase transition from a low-doped CdSe NC to Cu 2 Se. In other words, a NC already doped with Cu + is much more likely to take up additional Cu + and make a sharp transition to Cu 2 Se, albeit at the expense of another NC which has acquired none or relatively few dopants. This bias represents positive co-operativity between ‘sites’ on the same NC. When energetic aspects of such positive co-operative behaviour were included in a lattice site model (Methods section) [25] , we were able to simulate all our experimental observations ( Fig. 2b ). We started with an ensemble of CdSe NCs, each with 20 bivalent sites for Cu + . For the first doping event within any NC, the magnitude of the free energy change Δ G was assumed to be small, making it a low probability event. However, each doping event increased, by an amount Δ g , the free energy change resulting from subsequent doping on the same NC. Thus, it is energetically more and more favourable for a NC to incorporate Cu + ions. This simple model reproduced the strongly sigmoidal response of the NC ensemble to the added Cu + . There was an extended latent region during which only a tiny fraction of NCs made a transition to Cu 2 Se. Most of the NCs made a transition over a narrow window around a critical Cu + feed concentration. The simulations also reproduced the rise in the number of defects in the ensemble with increasing Cu + feed concentration. The number of defects reached a maximum around the critical concentration, following which it gradually decreased to zero. If there were no such positive co-operative bias (that is, if every site in the CdSe ensemble had a similar affinity for Cu + regardless of whether the site is on an already doped NC or an undoped one), the exchange process would be a diffusion-limited one. In such a case, each NC would exchange gradually via a continuum of intermediary CdSe/Cu 2 Se heterostructure states. The titration curve would be Langmuirian ( n H =1) rather than sigmoidal ( n H >1). Thus, a positive co-operative model, similar to one employed in biomacromolecular systems [26] , captures the observed behaviour of the cation exchange process. Nevertheless it still leaves open the question of the atomistic mechanism for co-operativity. In haemoglobin, oxygen binding at one of the heme subunits leads to a conformational change in the neighbouring subunits, which increases the affinity of the neighbour site for oxygen binding, a phenomenon known as allostery [22] . Allosteric coupling between lattice sites of a NC can originate from a few different structural factors. As described earlier, owing to charge compensation, Cu + doping results in the creation of Cd 2+ vacancies, one vacancy for every two interstitial Cu + impurities. These lattice vacancies provide hopping sites for enhanced in-diffusion of additional Cu + ions into the NC and out-diffusion of Cd 2+ ions from the NC. Second, the local negative polarization at a Cd 2+ vacancy site could electrostatically attract other positively charged Cu + ions. Third, inclusion of interstitial impurities and formation of vacancies would strain the NC lattice greatly enhancing the thermodynamic driving force for Cu + substitutions and structural transition to Cu 2 Se. Such mechanisms have been found to be operative in super-ionic solids [27] . Cation exchange with another common monovalent cation Ag + showed similar results: a sigmoidal titration curve and a maximum in the defect luminescence intensity around the critical concentration ( Fig. 5 ), indicating that the co-operative mechanism of cation exchange is not specific just to Cu + . The Ag system appears to be less co-operative than the Cu system: the titration curve is not as steep. The Hill fit shows a value of n H =3.2 smaller than for Cu + . The plot of the defect luminescence intensity as a function of feed concentration does not show a sharp peak, rather a plateau. Although the physical reason for this difference is not understood, it could be due to the significantly larger size of Ag + than Cu + . The larger Ag + ions may have a lower propensity to occupy interstitial sites and substitutional doping may be more prevalent than in the Cu + case. 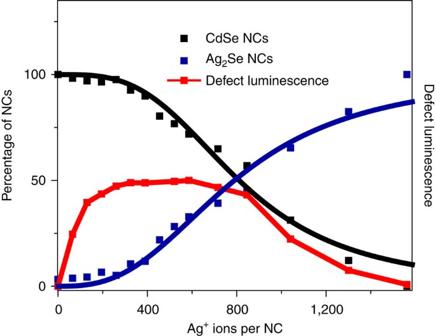Figure 5:Co-operativity in the cation exchange of CdSeNCs with Ag+. A plot of the fraction of NCs in the CdSe state (black dots) and those in the Ag2Se state (blue) as a function of added Ag+is sigmoidal, indicative of co-operative behaviour. Below a critical concentration of∼500 Ag+/NC, very few NCs undergo a transition to the Ag2Se state. A fit to the Hill plot (solid black line,R=0.973) yields a co-operativity factor ofnH=3.2. The fraction of NCs in the CdSe state was determined from the height of the CdSe excitonic peak and the fraction in the Ag2Se state was determined from the Ag2Se band-to-band absorption at 1.82 eV. The absorption and PL data is shown inSupplementary Fig. S5, and the procedure for analysis is described in Methods. The rise in the Ag2Se fraction tracks well with the drop in the CdSe fraction. The defect luminescence intensity (red), integrated across its broad band, increases as Ag+is added, until it reaches a maximum around the critical concentration, beyond which it decreases, until it reaches zero. Figure 5: Co-operativity in the cation exchange of CdSe NC s with Ag + . A plot of the fraction of NCs in the CdSe state (black dots) and those in the Ag 2 Se state (blue) as a function of added Ag + is sigmoidal, indicative of co-operative behaviour. Below a critical concentration of ∼ 500 Ag + /NC, very few NCs undergo a transition to the Ag 2 Se state. A fit to the Hill plot (solid black line, R =0.973) yields a co-operativity factor of n H =3.2. The fraction of NCs in the CdSe state was determined from the height of the CdSe excitonic peak and the fraction in the Ag 2 Se state was determined from the Ag 2 Se band-to-band absorption at 1.82 eV. The absorption and PL data is shown in Supplementary Fig. S5 , and the procedure for analysis is described in Methods. The rise in the Ag 2 Se fraction tracks well with the drop in the CdSe fraction. The defect luminescence intensity (red), integrated across its broad band, increases as Ag + is added, until it reaches a maximum around the critical concentration, beyond which it decreases, until it reaches zero. Full size image Although positive co-operativity between sites of individual NCs explains all our observed results, a related mechanism is worth considering. It is possible for initial Cu (or Ag) impurities formed within a NC to cluster together into a critical-size nucleus, initiating spontaneous growth of the Cu 2 Se (or Ag 2 Se) phase within the NC. This is reminiscent of the photographic development of silver iodide, where a latent four-atom nucleation cluster triggers rapid spontaneous growth of Ag [28] , [29] , [30] . Such a nucleation–growth mechanism could give rise to the observed two-state behaviour and the sharp sigmoidal transition. However, the topotactic nature of cation exchange [31] is not compatible with a nucleation-driven mechanism. In the latter mechanism, the final nanostructure morphology would be dictated by the growing nucleus, rather than by the starting ionic template. A common feature across many co-operative systems is that each binding event pre-organizes other sites for binding, thereby reducing the number of non-productive configurations and resulting in greatly enhanced reaction rates. For instance, co-operativity allows a protein to fold rapidly within milliseconds, rather than requiring the protein to sample all possible configurations. The latter would need a time longer than the age of the universe. It is possible that cation exchange reactions in NCs are driven to completion due to the strongly co-operative nature of the transition. Akin to co-operativity between molecular units in the biological world, co-operativity between atoms may be ubiquitous in the solid state, where there is no dearth of multi-site systems. Formation of defects, interfaces or strain may provide the required inter-site interactions. Co-operative behaviour in solid-state systems needs closer attention, especially in relation with closely linked processes such as phase transitions and nucleation [32] , [33] and due to the utility of co-operative phenomena in predicting and controlling materials’ transformation outcomes. Nonlinear behaviour induced by co-operativity may allow the design of sensors with tight regulation. Synthesis of CdSe NCs The procedure for synthesis of CdSe NCs was adapted from Manna and co-workers [34] . Three grams of trioctylphosphine oxide, 0.280 g of octadecylphosphonic acid (ODPA) and 0.060 g of cadmium oxide were mixed in a 25 ml three neck flask, heated to 150 °C and exposed to vacuum for 1 h. Under argon, the solution was heated to 320 °C and held at that temperature until the solution was optically clear, indicating complete dissolution of cadmium oxide. At this point, 1.5 g of tri- n -octylphosphine (TOP) was injected into the flask. The flask was heated to 370 °C and a TOP-Se solution (0.058 g of selenium powder and 0.360 g of TOP) was injected into the flask. The reaction time was 1 min for obtaining CdSe NCs of 4 nm diameter. After the synthesis, the NCs were repeatedly precipitated with methanol followed by re-dissolution in toluene. Stoichiometry calculations for cation exchange titrations For titrations, the initial concentration of Cd 2+ ions from the CdSe NCs in each reaction cuvette was determined. From the position of the first exciton, λ , the diameter, D , of the NC and the extinction coefficient were calculated using the equations [35] : The NCs used in all the titrations had a diameter of ∼ 4 nm. The extinction coefficient and the absorbance at the first exciton were used to determine the concentration of NCs. From the diameter, the volume and mass of NCs was calculated, from which the total mass and molar amount of Cd 2+ ions in each CdSe NC solution was determined. All titrations were done with approximately equal concentrations of CdSe NCs. Each Cu + titration involved 4.8 × 10 −6 mol of Cd 2+ ions being exchanged with one stoichiometric equivalent of Cu + ions (9.6 × 10 −6 mol of Cu(I)PF 6 ) dissolved in 200 μl of methanol. The details for each incremental addition in the titration is given in Supplementary Table S2 . The right-most column of this table was used as the x axis value for the titration plots shown in Fig. 2 . Cation exchange procedure All exchange reactions were carried out in septa-capped 3.5 ml quartz cuvettes. In an oxygen and moisture-free glove box, CdSe NCs were dispersed in 3.0 ml of toluene. Initial Cd 2+ molar amounts were calculated as described above to be 4.8 × 10 −6 mol Cd 2+ . In total, 9.6 × 10 −6 mol of tetrakis(acetonitrile)copper(I) hexafluorophosphate (Cu(I)PF 6 ) in 200 μl of methanol was added during each titration. NC samples were prepared in the glove box in air-free conditions and kept in air-free cuvettes during the exchange reactions. Additions took place outside of the glove box. A solution of Cu(I)PF 6 in methanol, prepared in the glove box and kept sealed during the experiment, was sequentially added to the reaction cuvette with a microliter syringe, taking care that the solution or sample were not exposed to air. Samples were stirred vigorously after each addition and the solution was allowed to equilibrate while stirring for ∼ 1 h, which is a time much in excess of the typical reaction time for complete cation exchange (<1 s). Absorption and photoluminescence (PL) spectra were then taken. Optical spectroscopy measurements Absorption spectra of exchanged CdSe NCs were collected on a Shimadzu UV-3600 scanning spectrophotometer with a 1 nm step size with toluene as a reference solvent. PL spectra of NCs were taken in toluene on a Cary Eclipse fluorimeter. Spectra were taken in the 650–900 nm wavelength range, where defect luminescence appears. All PL measurements were performed using the same slit width (5 nm), scan speed (120 nm/min), excitation wavelength (450 nm) and photomultiplier tube voltage. Analysis of absorption and PL spectra The total volume change over the entire titration was <10%, therefore correction of spectra for volumetric dilution was not necessary. The acquired absorbance spectra contain absorption from both unexchanged CdSe NCs and formed Cu 2 Se NCs. The absorption contribution of the formed Cu 2 Se NCs was subtracted from the acquired spectra to isolate the absorption of unexchanged CdSe NCs as follows: Here, we use the fact that at 1.82 eV, the absorption contribution from CdSe is negligible. The absorbance A at the first exciton peak of the corrected spectrum is proportional to the concentration of unexchanged CdSe NCs in solution as per Beer–Lambert’s law. This absorbance A normalized to a value of 100% at 0% exchange is equal to the percentage of CdSe NCs that is still unexchanged. This percentage was plotted as a function of Cu + added in Fig. 2a . The absorbance of Cu 2 Se at 1.82 eV (that is, above its bandgap absorption onset) can be used to estimate the relative concentration of Cu 2 Se NCs produced over the course of the titration. The absorbance at 1.82 eV normalized to a value of 100% at full exchange is equal to the percentage of Cu 2 Se NCs formed. This percentage was also plotted in Fig. 2a as a function of Cu + feed concentration. PL spectra were corrected by removing the contribution from the excitonic PL of CdSe NCs as follows: After this correction, the defect luminescence bands were integrated between 650 and 900 nm. The integrated defect PL signal was plotted in Fig. 2a as a function of Cu + feed concentration. We also performed a control experiment to confirm that methanol exposure alone does not give rise to defect PL in the NCs ( Supplementary Fig. S3 ). Electron microscopy High-resolution transmission electron microscopy (HRTEM) images were taken using a JEOL 2010 LaB 6 operating at 200 kV. High-angle annular dark-field scanning electron transmission microscopy (HAADF-STEM) images were acquired on a JEOL 2010F at 200 kV with a 0.5 nm size beam. Samples of NCs were prepared by drop-casting NCs in toluene on an ultrathin carbon grid followed by repeated washing with methanol. NC morphology HRTEM and HAADF-STEM images ( Supplementary Figs S4 and S5 ) show the morphology of NCs as a function of the feed Cu + concentration in Cu + ions per NC. Samples were made from adding Cu(I)PF 6 in 200 μl methanol to CdSe NCs in toluene. The NCs were drop-casted from this toluene:methanol mixture onto a Cu grid, followed by washing with methanol to remove excess Cu + and Cd 2+ resulting from exchange. Images show preservation of size and morphology throughout the exchange process. NC sizing analysis was performed on HAADF-STEM images. Lattice fringes in HRTEM show that NCs maintain crystallinity throughout the exchange process. Elemental analysis ICP-OES (inductively coupled plasma optical emission spectrometry) was performed on a Perkin-Elmer Optima 2000 DV instrument. To prepare samples, NCs were repeatedly washed and precipitated with methanol to remove excess ions in solution. Approximately 1 mg of each sample was digested with 16 M HNO 3 and subject to ICP-OES analysis for determination of the molar ratios of Cd, Cu and Se ( Supplementary Table S1 ). Exchange with Ag + Titration experiments with Ag + were performed in an identical manner as those with Cu + . Initial Cd 2+ molar amounts were calculated as described above to be 4.4 × 10 −6 mol of Cd 2+ in each cuvette. In total, 8.9 × 10 −6 mol of silver nitrate (AgNO 3 ), corresponding to one stoichiometric equivalent, was the calculated amount to be added over the entire titration Slightly more was actually found to be needed (1.1 × 10 −5 mol of AgNO 3 in 240 μl of methanol) to ensure complete disappearance of the first exciton peak of CdSe. Absorption and PL spectra were corrected and processed using the same methods described earlier. Uncorrected absorption spectra ( Supplementary Fig. S6a ) were baseline corrected ( Supplementary Fig. S6c ) to account for absorption of Ag 2 Se NCs. The CdSe exciton peak heights were then analysed to estimate the percentage of NCs exchanged as a function of Ag + added ( Fig. 5 ). The PL spectra ( Supplementary Fig. S6b ) were corrected ( Supplementary Fig. S6d ) to remove the band-edge PL. Following correction, the defect luminescence band was integrated to obtain the trend in defect luminescence intensity as a function of Ag + added ( Fig. 5 ). X-ray photoelectron spectroscopy XPS analysis was performed on NCs exchanged with 0, 325 and 651 Cu + ions per NC. A Kratos Axis ULTRA instrument was used, which uses a monochromatized Al K α X-ray source of 15 kV ( ∼ 10 mA). The instrument consisted of separate specimen transfer and analysis chambers, typically operated at 5E−07 and 1E−09 Torr, respectively. The Cu 2p 3/2 spectrum was fitted with 30% Gaussian/70% Lorentzian peak shapes. C 1s peak was used as a reference. The samples subject to 325 and 651 Cu + ions per NC ( Fig. 4b and Supplementary Fig. S1c respectively) show a Cu 2p 3/2 with a fitted peak position of 932.5 eV, which suggests a 1+ oxidation state. To distinguish between Cu 0 and Cu + , high-resolution spectra were collected around the X-ray-induced Cu LMM Auger peak (shown in Fig. 4c and Supplementary Fig. S1d ). The peak position of 917.2 eV (K.E.) corresponds to Cu (1+) . The absence of the Cu (1+) peak in the Cu 2p 3/2 ( Supplementary Fig. S1a ) and Cu LMM ( Supplementary Fig. S1b ) spectra for the unexchanged sample confirms that there is no Cu in the original CdSe NCs. Theoretical model We simulated the response of NCs using a lattice-site model. Each NC was assumed to have a size of n =20 sites, each of which can incorporate two Cu + ions. Co-operativity was introduced in this model by requiring that doping takes place sequentially: only when a doping event has taken place at the first site in the NC does a second site become available in that NC, and so on. here M , ML , ML 2 and so on are relative concentrations of NC complexes from CdSe through to Cu 2 Se and k 1 , k 2 , k 3 and so on are association constants for each sequential doping step. We assumed that the association constant of the first doping event k 1 has a relatively small magnitude (10 −2 M −1 ). However, the first step enhances the free energy for the second step by an amount Δ g , and the second step enhances that of the third one and so on. Therefore, or, where a =exp −Δ g/kT . As Δ g is negative, a is a positive integer, which we term as the interaction parameter. The magnitude of a depends directly on the magnitude of free energy stabilization (Δ g ) relative to thermal energy ( kT ). For instance, a 0.1-eV stabilization can result in a ∼ 55, which was a typical value used in the simulations. A higher value of a would allow the transition to be achieved over a narrower concentration window for the same value of k 1 . For a free Cu + concentration c and Cd 2+ concentration d , concentrations of the different NC complexes can be given in terms of the concentration of unexchanged CdSe NCs M as: In general, where we define a dimensionless k : The fraction of NCs in the pure CdSe state is given by: where The fraction of NCs in the Cu 2 Se state is given by: 1- ML n / M T gives the fraction of NCs that are either purely CdSe or Cu-doped CdSe. The total concentration of Cu + dopants is given by: Note in the above expression Cu + ions in Cu 2 Se state are not included as they are no longer in the form of dopants and do not contribute to defect luminescence. Free Cu + ions in solution are not included either. c d is also equal to two times the concentration of Cd 2+ vacancies. The concentration of Cu + incorporated in the NCs, including in the form of Cu 2 Se, is given by: The free Cd 2+ concentration is given by: The free Cu + concentration is given by: and the total Cu + concentration as: How to cite this article: White, S.L. et al. Co-operativity in a nanocrystalline solid-state transition. Nat. Commun. 4:2933 doi: 10.1038/ncomms3933 (2013).